Revealing a double-inversion mechanism for the F−+CH3Cl SN2 reaction Stereo-specific reaction mechanisms play a fundamental role in chemistry. The back-side attack inversion and front-side attack retention pathways of the bimolecular nucleophilic substitution (S N 2) reactions are the textbook examples for stereo-specific chemical processes. Here, we report an accurate global analytic potential energy surface (PES) for the F − +CH 3 Cl S N 2 reaction, which describes both the back-side and front-side attack substitution pathways as well as the proton-abstraction channel. Moreover, reaction dynamics simulations on this surface reveal a novel double-inversion mechanism, in which an abstraction-induced inversion via a FH···CH 2 Cl − transition state is followed by a second inversion via the usual [F···CH 3 ···Cl] − saddle point, thereby opening a lower energy reaction path for retention than the front-side attack. Quasi-classical trajectory computations for the F − +CH 3 Cl( ν 1 =0, 1) reactions show that the front-side attack is a fast direct, whereas the double inversion is a slow indirect process. Bimolecular nucleophilic substitution (S N 2) reactions play a fundamental role in chemistry; therefore, many experimental and theoretical studies have focused on the atomic-level dynamics and mechanism of this class of reactions [1] , [2] , [3] , [4] , [5] , [6] , [7] , [8] , [9] . In a typical S N 2 reaction, X − +H 3 CY→XCH 3 +Y − , the reactive events usually begin with a back-side attack forming a pre-reaction complex, which can be either a hydrogen-bonded X − ···HCH 2 Y or a traditional ion-dipole X − ···H 3 CY complex, then the system goes through a central transition state (TS), where a new X−C bond forms and the C−Y bond breaks while the umbrella motion of the CH 3 unit inverts the configuration around the tetrahedral carbon centre. This is the famous Walden inversion mechanism of S N 2 reactions, which is described in every organic chemistry textbook. An important feature of this mechanism is its stereo-specificity, which means that an inversion always occurs resulting in a specific configuration of the product molecule, which is the opposite of the reactant’s configuration. Stereo-specificity has exceptional importance in nature, for example, all the natural amino acids exist in a specific configuration and their stereo-isomers (enantiomers) cannot be found in natural proteins. So far, we have thought that the stereo-chemistry of the S N 2 reactions is well-understood. Besides the well-known Walden inversion mechanism, there is a front-side attack pathway, which goes over a high energy barrier and results in retention of configuration. This front-side attack mechanism is much less studied than the Walden inversion [10] , [11] , [12] , [13] . Due to the high barrier of the former, the S N 2 reactions are known to proceed via Walden inversion at low collision energies ( E coll ) and the front-side attack pathway may open at higher E coll . Note that one may distinguish between direct rebound and stripping, as well as indirect (ion-dipole and/or hydrogen-bonded complex formation, roundabout and barrier recrossing) mechanisms [14] , but in the present study we consider these as variants of the back-side attack inversion mechanism. Here we perform high-level reaction dynamics simulations for the F − +CH 3 Cl prototypical S N 2 reaction using a new ab initio global potential energy surface (PES). Since in a simulation one can label the three H atoms, we can examine the configurations of the CH 3 F products. As expected, we find that most of the CH 3 F molecules have inverted configurations. However, some of the trajectories result in retention of configuration, which is very surprising, because this is found at low E coll well below the barrier height of the front-side attack pathway. How can this happen? In what follows, we describe the details of the reaction dynamics computations and reveal a novel mechanism for S N 2 reactions. Potential energy surface Reaction dynamics simulations require the knowledge of the PES, which governs the motion of the atoms in a chemical reaction [15] , [16] , [17] . Full-dimensional analytical PESs that describe both the back- and front-side attack mechanisms have not been developed for S N 2 reactions. Following our previous work [9] , here we report a global PES for the F − +CH 3 Cl reaction by fitting about 52,000 high-level ab initio energy points (see Supplementary Methods ). As Fig. 1 shows, the PES describes the back and front-side attack substitution pathways, as well as the abstraction channel leading to HF+CH 2 Cl − . Furthermore, we have uncovered another pathway, which begins with an abstraction-induced inversion via a TS of C s symmetry followed by a second inversion via the usual C 3v TS. We call this as a double-inversion mechanism, which results in the retention of configuration. It is also possible that the first induced inversion is not followed by a reactive substitution event; thus, the collision results in an inverted reactant. 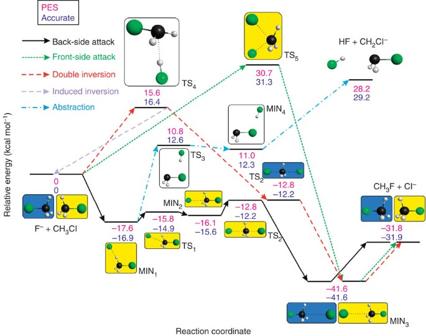Figure 1: Schematic of the global potential energy surface (PES) of the F−+CH3Cl reaction. Arrows show the different stereo-specific reaction pathways leading to retention (yellow) and inversion (blue) of the initial configuration (yellow). The accurate benchmark energies and the PES values are relative to F−+CH3Cl(eq). Figure 1: Schematic of the global potential energy surface (PES) of the F − +CH 3 Cl reaction. Arrows show the different stereo-specific reaction pathways leading to retention (yellow) and inversion (blue) of the initial configuration (yellow). The accurate benchmark energies and the PES values are relative to F − +CH 3 Cl(eq). Full size image Characterization of the stationary points We have characterized the stationary points of the PES by a sophisticated composite focal-point analysis (FPA) [18] approach considering extrapolation to the complete basis set limits, electron correlation beyond the ‘gold-standard’ CCSD(T) method, correlation of all the electrons (core and valence) and scalar relativistic effects. More details about the FPA are given in Supplementary Methods . As Fig. 1 shows, the relative energies corresponding to the fitted analytical PES agree well, usually within 1 kcal mol −1 , which is considered as ‘chemical accuracy’, with the benchmark FPA data. The F − +CH 3 Cl S N 2 reaction is highly exothermic, Δ E e =−31.9 kcal mol −1 , whereas the abstraction channel is endothermic, Δ E e =29.2 kcal mol −1 . The analytical PES accurately describes many minima (complexes) and saddle points (transitions states) that separate the reactants from the products. The back-side attack substitution pathway goes through H-bonded C s and ion-dipole C 3v F − ···CH 3 Cl complexes, a C 3v [F···CH 3 ···Cl] − TS and a C 3v FCH 3 ···Cl − complex, which are all below the F − +CH 3 Cl(eq) asymptote by 16.9 kcal mol −1 , 15.6 kcal mol −1 , 12.2 kcal mol −1 and 41.6 kcal mol −1 , respectively, whereas the front-side attack substitution has a high classical barrier of 31.3 kcal mol −1 . Furthermore, we have found a TS for the double-inversion mechanism as shown in Fig. 1 , which opens a substantially lower energy configuration-retaining pathway with a classical barrier height of 16.4 kcal mol −1 than the front-side attack mechanism. Structures and harmonic vibrational frequencies of all the stationary points can be found in the Supplementary Tables 1–4 . Reaction dynamics simulations With an accurate full-dimensional analytical PES at hand, we can go much further than predicting reaction mechanisms based on stationary points. We have performed quasi-classical trajectory (QCT) computations on the PES, thereby following the motion of the atoms along the reaction path. We have run about four million trajectories for the ground-state and symmetric-CH-stretching-excited F − +CH 3 Cl( ν 1 =0, 1) reactions (the initial conditions and analysis techniques are described in Supplementary Methods ). Integral cross-sections Integral cross-sections (ICSs) as a function of E coll are shown in Fig. 2 . Since the exothermic back-side attack substitution reaction does not have a barrier, the S N 2 ICSs are large and decrease steeply with E coll . The H-abstraction reaction is highly endothermic, its zero-point energy (ZPE) corrected reaction enthalpy is 24.5 kcal mol −1 on the PES, and the abstraction saddle point is well below the product asymptote. The ICSs show that the HF+CH 2 Cl − channel opens as soon as it becomes energetically available and the ICSs increase with E coll . (The small reactivity at E coll <24.5 kcal mol −1 is due to ZPE violation of the products.) The ν 1 =1 excitation has only slight effect on the S N 2 reactivity, showing that the CH symmetric stretching vibrational mode behaves as a spectator in the back-side attack S N 2 reaction. In the case of the H-abstraction, as expected, CH stretching excitation substantially enhances the reactivity and lowers the reaction threshold. It is interesting to find that the ν 1 =1 abstraction ICSs increase up to a E coll of ~40 kcal mol −1 and then a slight decay is seen, because the faster reactants have less time to interact with each other. This depression of reactivity with the increase of E coll was also found in the H+CD 4 →HD+CD 3 reaction [19] . 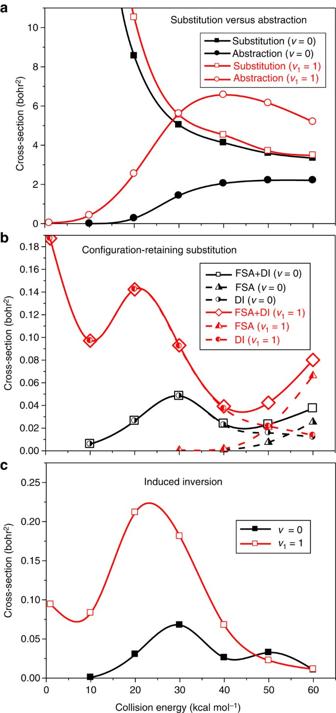Figure 2: Cross-sections as a function of collision energy for the ground-state and CH-stretching-excited F−+CH3Cl(ν1=0, 1) reactions. (a) back-side attack substitution (Cl−+CH3F) and abstraction (HF+CH2Cl−) channels, (b) retention of configuration via front-side attack (FSA) and double-inversion (DI) substitution mechanisms and (c) induced inversion of the reactant CH3Cl. Figure 2: Cross-sections as a function of collision energy for the ground-state and CH-stretching-excited F − +CH 3 Cl( ν 1 =0, 1) reactions. ( a ) back-side attack substitution (Cl − +CH 3 F) and abstraction (HF+CH 2 Cl − ) channels, ( b ) retention of configuration via front-side attack (FSA) and double-inversion (DI) substitution mechanisms and ( c ) induced inversion of the reactant CH 3 Cl. Full size image Figure 2 also shows the ICSs for the configuration-retaining substitution. These ICSs are much smaller than those of the inversion mechanism (1.1% and 2.3% at E coll =60 kcal mol −1 for ν =0 and ν 1 =1, respectively), but the absolute ICSs are not negligible since, for example, the H+CD 4 reaction has similar small ICSs [19] . For F − +CH 3 Cl( ν =0), the configuration-retaining pathway opens at a E coll of ~10 kcal mol −1 , the ICSs rise up to E coll =~30 kcal mol −1 , then decay and increase again around E coll =40−50 kcal mol −1 . The adiabatic barrier height for the front-side attack path is 29.3 kcal mol −1 on the PES; thus, this mechanism cannot produce CH 3 F with retention of configuration in the 10−30 kcal mol −1 E coll range. Examination of many configuration-retaining trajectories has revealed a double-inversion mechanism, which has an adiabatic barrier height of only 12.6 kcal mol −1 on the PES, thereby allowing retention of configuration at E coll where the front-side attack pathway is closed. Based on the analysis of the integration time of the reactive trajectories, we have found that none of the double-inversion trajectories finished within 0.65 ps, whereas all the front-side attack reactions occurred faster than 0.65 ps. Thus, on the basis of the integration time we could distinguish between double-inversion and front-side attack trajectories and we could get the mechanism-specific retention ICSs as shown in Fig. 2 . As expected, at low E coll every configuration-retaining substitution event goes via double inversion. The front-side attack pathway opens at a E coll of ~40 kcal mol −1 , well above the adiabatic barrier. Now we can explain the E coll dependence of the ICSs: the ICSs start to increase when the double-inversion pathway opens, above E coll of 30 kcal mol −1 the reactivity via double inversion decreases, because the large E coll does not favour the indirect mechanism and the abstraction channel opens, then at E coll =~40 kcal mol −1 the front-side attack reactions raise the ICSs again. After the discovery of the double-inversion mechanism, we can also expect to get inverted CH 3 Cl molecules if the first inversion is not followed by substitution. Indeed, the analysis of the ‘non-reactive’ trajectories revealed that some of the reactants became inverted via an abstraction-induced inversion. As Fig. 2 shows, the E coll dependence of the induced-inversion ICSs is consistent with that of the double-inversion ICSs: the induced inversion opens above E coll =~10 kcal mol −1 and the ICSs have a maximum at E coll =~30 kcal mol −1 . Since the first step of the double- and induced-inversion mechanisms is pulling out a proton, CH-stretching excitation substantially enhances the double and induced inversions and diminishes their energy thresholds. Differential cross-sections Angular distributions for the F − +CH 3 Cl( ν 1 =0, 1) reactions at E coll =50 kcal mol −1 are shown in Fig. 3 . As seen, the scattering angle distributions are very different for the various mechanisms. The back-side attack pathway results in mainly backward scattered products, as expected, since the [F···CH 3 ···Cl] − TS is collinear and the direct rebound mechanism is dominant at a high E coll (refs 9 , 20 ). The front-side attack substitutions are also direct; thus, dominance of sideways scattering is seen as expected based on the TS structure, because the F−C−Cl angle is about 80° at the TS. The double-inversion substitutions result in more-or-less isotropic angular distributions indicating an indirect mechanism, where long-lived complexes are formed. For the H-abstraction channel, a clear preference for backward scattering is found, suggesting that stripping is not significant at E coll =50 kcal mol −1 . CH-stretching excitation virtually does not affect the angular distributions, perhaps the most significant effect is seen for the front-side attack, where ν 1 =1 excitation broadens the angular distributions. In Supplementary Fig. 1 , angular distributions are also shown at a smaller E coll of 30 kcal mol −1 . The shapes of the distributions are very similar at 30 and 50 kcal mol −1 E coll . Note that the front-side attack pathway is not open at the lower E coll . 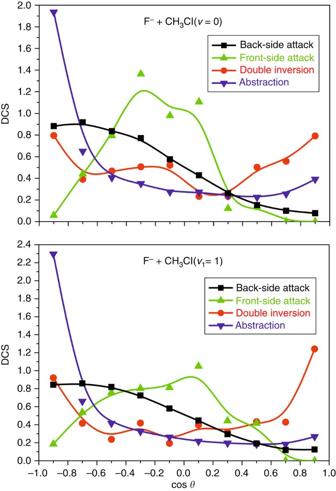Figure 3: Scattering angle distributions. Angular distributions of the ground-state and CH-stretching-excited F−+CH3Cl(ν1=0, 1) reactions for the back-side attack, double-inversion and front-side attack substitution pathways (Cl−+CH3F) and for the abstraction channel (HF+CH2Cl−) at a collision energy of 50 kcal mol−1. Each distribution is normalized to have the same unit area. Figure 3: Scattering angle distributions. Angular distributions of the ground-state and CH-stretching-excited F − +CH 3 Cl( ν 1 =0, 1) reactions for the back-side attack, double-inversion and front-side attack substitution pathways (Cl − +CH 3 F) and for the abstraction channel (HF+CH 2 Cl − ) at a collision energy of 50 kcal mol −1 . Each distribution is normalized to have the same unit area. Full size image Retention pathways step by step Representative trajectories illustrating the key steps of the front-side attack and the double-inversion mechanisms, and showing the potential energy as a function of time are shown in Fig. 4 . As seen, in the first 0.15 ps while the reactants approach each other, the potential energy oscillates around 12 kcal mol −1 , which corresponds to half of the ZPE of CH 3 Cl, in agreement with the virial theorem. The front-side attack substitution is very direct, the system goes through a high barrier and vibrationally excited CH 3 F product is formed. The double inversion occurs on a much longer time scale. First, the F − abstracts a proton (H + ), but the system does not have enough energy to fall apart, thus HF starts to move around CH 2 Cl − and eventually a C−H bond forms again while the configuration around the carbon centre gets inverted. Second, a C−F bond forms and the C−Cl bond breaks resulting in a second inversion via the usual C 3v TS. Therefore, the double inversion results in retention of configuration via a long indirect mechanism. These unusual reaction pathways were verified by direct ab initio computations along selected trajectories. As shown in Fig. 4 , the ab initio data reproduce remarkably well the energies obtained from the analytically fitted PES, thereby confirming the new findings. 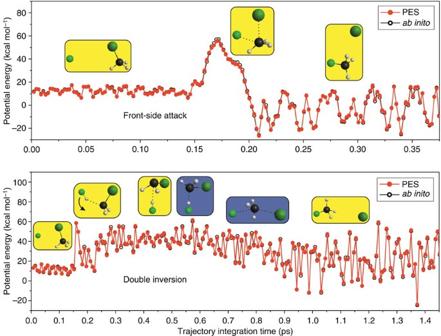Figure 4: SN2 retention mechanisms. Snapshots of representative trajectories showing the front-side attack and double-inversion mechanisms of the F−+CH3Cl(ν=0) reaction at a collision energy of 50 kcal mol−1. The potential energies, relative to F−+CH3Cl(eq), obtained from the fitted PES and directab initiocomputations are shown as a function of time. Blue background denotes an inverted configuration relative to that of the reactant (yellow). Figure 4: S N 2 retention mechanisms. Snapshots of representative trajectories showing the front-side attack and double-inversion mechanisms of the F − +CH 3 Cl( ν =0) reaction at a collision energy of 50 kcal mol −1 . The potential energies, relative to F − +CH 3 Cl(eq), obtained from the fitted PES and direct ab initio computations are shown as a function of time. Blue background denotes an inverted configuration relative to that of the reactant (yellow). Full size image The double-inversion mechanism revealed here for the F − +CH 3 Cl reaction may be a general pathway for substitution reactions, where hydrogen/proton abstraction is a competing channel. We plan to develop analytical global PESs for other systems to see if this is the case. Furthermore, it is important to note that the first step of the double inversion is reminiscent of the famous roaming mechanism discovered for the photo-dissociation of formaldehyde (H 2 CO) [21] . In roaming, the radical fragments, H···HCO, do not have enough energy in the dissociation coordinate to break apart; therefore, they follow a non-traditional path to form the molecular products, H 2 +CO. In double inversion, the FH···CH 2 Cl − complex cannot dissociate, but the system has enough energy to invert the configuration around the carbon atom, thereby opening a new way for retention in S N 2 reactions. The roundabout S N 2 mechanism also has features similar to roaming [14] ; therefore, the present study may inspire future research to focus on the possibility of retention via the roundabout pathway and the abstraction-induced mechanisms in S N 2 reactions. It is possible that the new double-inversion mechanism could be related with the already known roundabout mechanism. Since the first step of the double inversion is an abstraction-induced inversion, the reaction may result in an inverted reactant molecule as shown in the present study. Finding inverted reactants could be a signature for the double-inversion mechanism. Finally, one should note that the above atomistic mechanisms are defined based on classical dynamics. This approach is usually a good approximation for chemical reactions, but, of course, the nuclei do not exactly follow a defined trajectory. A time-dependent quantum mechanical treatment of the nuclear dynamics could show the regions of the configuration space in which the wave functions have non-negligible values. The comparison of the present findings with future quantum dynamical results may add to our understanding of chemical reaction mechanisms. Potential energy surface The global analytical full-dimensional PES for the F − +CH 3 Cl reaction is obtained by fitting 52,393 ab initio energy points computed by an efficient composite method. We have selected structures that cover the configuration space and energy range of chemical importance. The composite ab initio energies are computed as where in parenthesis the core correlation energy increment is given as a difference between all-electron (AE) and frozen-core (FC) energies. This composite method provides AE-CCSD(T)/aug-cc-pCVQZ quality results within a root-mean-square error of only 0.35 kcal mol −1 . The analytical representation of the PES is obtained by a fifth-order fit using the permutationally invariant polynomial approach [15] , [16] based on Morse-like variables, exp(– r ij / a ), where r ij are the inter-atomic distances and a =3 bohr. The linear least-squares fit, with weight of E 0 /( E + E 0 ), where E 0 =31 kcal mol −1 and E is relative to the global minimum, provides 3,313 coefficients. These coefficients are provided in Supplementary Data 1 . The root-mean-square fitting errors are 0.31 kcal mol −1 , 0.51 kcal mol −1 and 1.38 kcal mol −1 for the energy ranges 0–31 kcal mol −1 , 31–63 kcal mol −1 and 63–157 kcal mol −1 , respectively. Benchmark ab initio thermochemistry The best technically feasible relative energies for the stationary points of the F − +CH 3 Cl reaction are obtained by the FPA [18] approach. First, we compute the structures and harmonic frequencies at the AE-CCSD(T)/aug-cc-pCVQZ and FC-CCSD(T)/aug-cc-pVTZ levels of theory, respectively, for all the minima and saddle points shown in Fig. 1 , except for TS 3 , TS 4 , TS 5 and MIN 4 , where the structures are obtained at the AE-CCSD(T)/aug-cc-pCVTZ level. Second, the benchmark FPA relative energies are obtained by considering (a) extrapolation to the complete basis set limit using AE-CCSD(T)/aug-cc-pCV n Z ( n =Q(4) and 5) energies, (b) post-CCSD(T) correlation effects up to CCSDT(Q) based on AE-CCSDT/aug-cc-pCVDZ and FC-CCSDT(Q)/aug-cc-pVDZ energy computations and (c) scalar relativistic effects at the second-order Douglas–Kroll AE-CCSD(T)/aug-cc-pCVQZ level of theory. QCT calculations QCT computations are performed for the F − +CH 3 Cl( ν 1 =0, 1) reactions using the new analytical PES. The initial conditions for the trajectories are as follows: (a) standard normal mode sampling is used, (b) trajectories are run at E coll of 1, 10, 20, 30, 40, 50 and 60 kcal mol −1 , (c) the total number of ν =0( ν 1 =1) trajectories are 145,000 (145,000), 125,000(125,000), 85,000(95,000), 645,000(725,000), 85,000(95,000), 645,000(725,000) and 85,000(95,000) at the above E coll , respectively, and (d) the integration time step is 0.0726, fs and each trajectory is propagated until the maximum of the actual inter-atomic distances is 1 bohr larger than the initial one. We have found that basically no S N 2 trajectory violates the product ZPE; thus, the QCT analysis considers all the trajectories. The stereo-specific configurations of CH 3 Cl and CH 3 F are analyzed based on the procedure described in ref. 22 . How to cite this article: Szabó, I. et al . Revealing a double-inversion mechanism for the F − +CH 3 Cl S N 2 reaction. Nat. Commun. 6:5972 doi: 10.1038/ncomms6972 (2015).